Electronically stabilized nanowire growth Metallic nanowires show unique physical properties owing to their one-dimensional nature. Many of these unique properties are intimately related to electron–electron interactions, which have a much more prominent role in one dimension than in two or three dimensions. Here we report the direct visualization of quantum size effects responsible for preferred lengths of self-assembled metallic iridium nanowires grown on a germanium (001) surface. The nanowire length distribution shows a strong preference for nanowire lengths that are an integer multiple of 4.8 nm. Spatially resolved scanning tunneling spectroscopic measurements reveal the presence of electron standing waves patterns in the nanowires. These standing waves are caused by conduction electrons, that is the electrons near the Fermi level, which are scattered at the ends of the nanowire. One-dimensional (1D) electron systems have recently received much attention [1] , [2] , [3] , [4] , [5] , [6] , [7] , [8] , [9] . This interest is driven by the fact that these systems display a myriad of exciting physical phenomena, such as the quantization of conductance and spin and charge density waves [10] , [11] , [12] , [13] . Even more intriguing and exotic new physics emerges when electron–electron interactions are taken into account [5] , [6] , [7] , [8] , [9] , [10] , [11] , [12] . Unfortunately, true 1D electron systems are virtually impossible to realize. An elegant way to realize a quasi 1D electron system is by using a quantum mechanical break junction set-up [14] , [15] . Almost perfect linear, chains of atoms have been created in these experiments, all showing evidence for quantum conductance. The most viable examples involve the 5d -transition metals Au, Pt and Ir. However, a severe drawback of quantum mechanical break junction chains is their length being limited to only a few atoms. The aforementioned drawback can be overcome by growing self-organizing atom chains on semiconductor surfaces. These systems constitute the best candidates for model systems to study the exotic and intriguing phenomena of 1D electron systems. Fortunately, the heavy 5d -transition metals such as Pt and Au have a strong tendency to self-assemble into defect-free, straight, long and narrow nanowires on annealing, subsequent to deposition on semiconductor group IV (001) surfaces [16] , [17] , [18] , [19] , [20] , [21] , [22] , [23] . The Pt- and Au-induced nanowires, although different in nature, that is, in their structure [16] , [17] , [18] , [19] , [20] , [21] , [22] , share the property of being able to attain lengths of up to a few microns. Guided by the similarities in quantum transport between Ir on the one hand and Au and Pt on the other hand, we have investigated the self-organized growth of Ir on Ge(001) using scanning tunneling microscopy (STM) and spectroscopy in an attempt to expand the playground for 1D physics. The notion that quantum size effects (QSE) in the growth of thin metal films can lead to smooth films with magic thicknesses has already been recognized a few decades ago [24] , [25] , [26] , [27] . For obvious reasons, the underlying oscillations of the electron density of states cannot be measured for thin films. In contrast, the electron standing waves patterns in wires can be visualized directly. In addition, several years ago, Crain et al . [28] reported oscillations in the distribution of chain lengths of the Au/Si(553) system, which were interpreted in terms of the electronic scattering vectors at the Fermi surface of the surface states. These authors found clear evidence for end states showing enhanced density of states at the end atom, irrespective of chain length. Later, Shin et al . [29] also reported oscillations in the density of states for the Au/Si(553) system at low temperatures. These oscillations were explained in terms of charge density waves and were not present at room temperature. Both features are distinctly different from our report below. Here we report the first observation of oscillations of the electron density of states along Ir wires with preferred, quantized lengths of a multiple of 4.8 nm. Our experiments provide a direct insight in the intimate relation between growth and QSE and reveal that the growth of Ir nanowires is stabilized by an electronic effect. Scanning tunneling microscopy The Pt nanowires and the Au-induced nanowires on Ge(001) are prime examples of how self-organization can result in beautifully organized domains of regular and parallel 1D wires (see Fig. 1 ). The latter are oriented parallel to the dimer row directions, that is, along the <110> directions of a pristine Ge(001) surface. These domains can extend up to a micrometre with low-defect densities [16] . The separation of adjacent wires is well-defined and in both cases equal to 1.6 nm. Also, the surrounding parts of the surface, not covered with wires, are pretty regular except for the so-called α-terraces, which exhibit a high degree of disorder [16] . Encouraged by this success, we have tried to achieve a similar result for the intimately related 5d -transition metal Ir. All efforts ended in a disappointing result, even after lengthy exploration of the parameter space for annealing (temperature, anneal times, heating and cooling rates and so on). Without exception, a quite messy arrangement of short wires was obtained without a well-defined distance between the wires and quite disordered adjacent terraces, very much like the above mentioned α-terraces. In Fig. 1b,c , representative STM images are shown. We do observe Ir nanowires with a density that depends on the amount of pre-deposited Ir. In contrast to the cases of Pt and Au, these wires are oriented perpendicular to the substrate dimer row directions. Surprisingly, a zoom-in on the wire structure, as shown in the inset of Fig. 1b , reveals that the wire is composed of a well-ordered double chain running perpendicular to the direction corresponding to that of the dimer rows on the original, clean host terrace, which is still vaguely visible. The white protrusions are assigned as Ir atoms. The chains in the twin structure are separated by 0.57 nm and the periodicity along the chains amounts to 0.8 nm, that is, exactly twice the in-plane Ge distance. Judging from many images like this, there is no apparent reason why these wires could not extend over a very long distance. 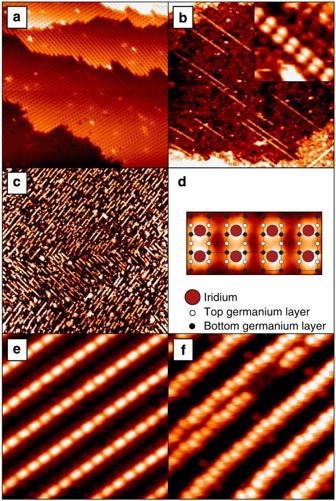Figure 1: STM images of self-organized nanowires on Ge(001). (a) STM image of Ge(001) before Ir deposition (−1.5 V, 0.5 nA image size is 35 × 35 nm2). (b) STM image after the deposition of 0.01 ML Ir and annealed at 450 K (−0.55 V, 0.5 nA, image size is 145 × 145 nm2. Inset: −0.86 V, 0.2 nA, image size is 4 × 4 nm2). (c) STM image after the deposition of 0.3 ML of Ir and annealed at 450 K (0.50 V, 0.5 nA, image size is 145 × 145 nm2). (d) Close up on an Ir nanowire. A simple ball and stick model for an Ir nanowire is superimposed on the STM image (−0.86 V, 0.2 nA). (e) STM image of an array of Pt nanowires on a Ge(001) surface (−1.5 V, 0.5 nA, image size is 8 × 8 nm2) and (f) STM image of an array of Au-induced nanowires on a Ge(001) surface (−1.5 V, 0.2 nA, image size is 7.5 × 7.5 nm2). Figure 1: STM images of self-organized nanowires on Ge(001). ( a ) STM image of Ge(001) before Ir deposition (−1.5 V, 0.5 nA image size is 35 × 35 nm 2 ). ( b ) STM image after the deposition of 0.01 ML Ir and annealed at 450 K (−0.55 V, 0.5 nA, image size is 145 × 145 nm 2 . Inset: −0.86 V, 0.2 nA, image size is 4 × 4 nm 2 ). ( c ) STM image after the deposition of 0.3 ML of Ir and annealed at 450 K (0.50 V, 0.5 nA, image size is 145 × 145 nm 2 ). ( d ) Close up on an Ir nanowire. A simple ball and stick model for an Ir nanowire is superimposed on the STM image (−0.86 V, 0.2 nA). ( e ) STM image of an array of Pt nanowires on a Ge(001) surface (−1.5 V, 0.5 nA, image size is 8 × 8 nm 2 ) and ( f ) STM image of an array of Au-induced nanowires on a Ge(001) surface (−1.5 V, 0.2 nA, image size is 7.5 × 7.5 nm 2 ). Full size image To understand why the Ir wires do not grow to huge lengths and to shed light on the obvious differences between Ir and Pt/Au, we show in Fig. 2 a histogram of the length distribution, obtained from 582 individual Ir nanowires. The histogram shows unequivocally an intriguing oscillation of the length of the wire with a period of about 4.8 nm. A strong preference for wires with a length of 4.8, 9.6 and 14.4 nm is clearly established, whereas indications for preferred lengths of about 19 and 23 nm are visible. We consider this as strong evidence for an electronic stabilization of the length of the nanowires. In other words, we suggest that quantum size interferences are responsible for the preferred lengths of the wires. Before discussing this feature and its consequences in more detail below, we first briefly discuss the basic features of quantum stability in thin metal films. We do note, in addition, that the periodicity of the length oscillations in Fig. 2 is 4.8 nm, that is, six elementary units of the nanowire. 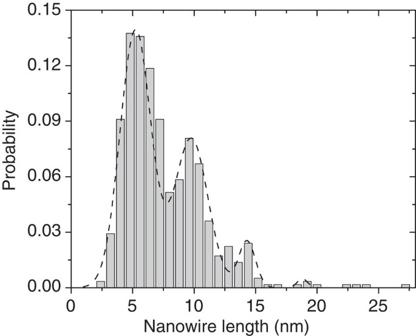Figure 2: Histogram of the length distribution of Ir nanowires. The dashed line serves as a guide to the eye. The Ir coverage was 0.3 ML. Figure 2: Histogram of the length distribution of Ir nanowires. The dashed line serves as a guide to the eye. The Ir coverage was 0.3 ML. Full size image Scanning tunneling spectroscopy The notion that QSE can affect the surface properties and stability of thin metal films on semiconductors or metals with a projected band gap dates back to 1976. The meeting of the condition for the presence of a standing wave pattern of the Fermi electrons between the interfaces, that is, quantum confinement, was found energetically favourable. Schulte [24] reported self-consistent electronic structure calculations that revealed thickness-dependent oscillations in the work function. Experimental evidence that QSE indeed affect epitaxial thin film growth has indeed been found by Hinch et al . [26] for Pb on Cu(111) and by Smith et al . [30] for Ag on GaAs(110). A preferred film thickness is obtained if the following condition applies: with λ F the Fermi wavelength, n d the number of layers with interatomic spacing . Another feature of electronic nature is the scattering of (Fermi) electrons by an isolated defect, a step edge or as in this case the end of a wire. This density modulation, which arises from an interference of incoming and reflected electron waves, has a periodicity of λ F /2 . This electron density modulation is referred to as a Friedel oscillation and is given by [31] , [32] , where k F is the Fermi wave vector, the background electron density, δ a phase factor, A the amplitude of the Friedel oscillation, D the dimension of the electron system and r the position with respect to the defect or impurity. The phase factor is closely related to charge spilling that occurs because of a non-perfect meeting of condition (1). Zhang et al . [27] pointed out that in principle three effects: quantum confinement size interference, charge spilling and Friedel oscillations contribute to the eventual thermodynamic stability of a thin film. Jia et al . [33] strongly suggested that Friedel oscillations can contribute to the stability of, in particular, thin Pb films in an anomalous fashion. The main access road to these Friedel oscillations in a film is through calculations. Experimentally, direct access is impossible, but QSE have been observed in electron reflectivity for electrons above the vacuum level, both in integral measurements [34] , [35] , [36] and in position-resolved experiments [37] , [38] , [39] , [40] , [41] . However, because of their unique geometry, the Ir wires would offer a unique and viable opportunity to access the relationship between size selection and Friedel oscillations in a most direct manner. This is further corroborated by the fact that Friedel oscillations decay very slowly in a 1D system. However, first we have to demonstrate that the Ir wires are metallic. In Fig. 3 , the differential conductivities of the Ir nanowires and the surrounding terraces are shown. The curve is the result of averaging over a number of long nanowires, which emerged at low Ir coverage (see Fig. 1b ). In contrast to the surrounding terraces, the Ir nanowires exhibit clearly a non-vanishing density of states at the Fermi level, indicating that they are metallic indeed. At 0.3–0.35 eV below the Fermi level, a pronounced electronic state is observed in the density of states of the nanowires. Despite the fact that this electronic state is located on the nanowires, thermal and instrumental broadening are too large to resolve the exact dimensionality from the energy dependence of the density of states [17] . 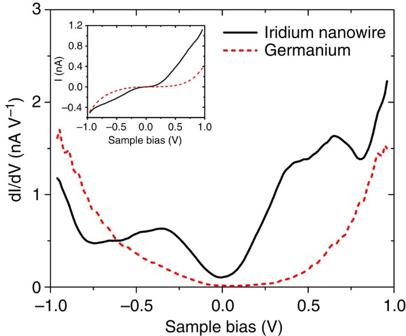Figure 3: Differential conductivity versus sample bias for the Ir nanowires and the clean Ge(001) surface. Solid line: Ir nanowires. The solid curve was obtained after averaging over a number of long nanowires (cf.Fig. 1b). Dashed line: Ge(001). Inset: corresponding I–V curves. Figure 3: Differential conductivity versus sample bias for the Ir nanowires and the clean Ge(001) surface. Solid line: Ir nanowires. The solid curve was obtained after averaging over a number of long nanowires ( cf . Fig. 1b ). Dashed line: Ge(001). Inset: corresponding I–V curves. Full size image After having fulfilled the two necessary requirements, that is, systematic size preferences and a non-zero density of states at the Fermi level, the crucial experiment is to measure the real space density of states across the nanowires and to relate its anticipated oscillatory nature to the preferred length of the wires. In Fig. 4a,b , the spatial variation of the density of states along the nanowires at the Fermi level is shown. An Ir nanowire with a length of L =4.8 nm exhibits one well-defined local density of states maximum at L/2 , whereas an Ir nanowire of length L =9.6 nm displays two maxima at L/4 and 3L/4 and a node at L/2 , respectively. In Fig. 4c , the spatial variation of the density of states recorded at 0.275 eV below the Fermi level for the 9.6-nm long Ir nanowire from Fig. 4b is shown. The differential conductivities are extracted from the I–V traces that were also used for the graph in Fig. 4b . The density of states reveals two minima at the ends of the nanowire and a maximum in the middle of the wire. It therefore carries the characteristic signature of an n= 1 state. On the basis of these experimental observations, we estimate that the bottom of the energy band is located around 360 meV below the Fermi edge, which is in good agreement with the local density of state curve depicted in Fig. 3 . These results show unambiguously that the observed size preference has its origin in an electronic effect: quantum size stabilization of preferred lengths of multiples of 4.8 nm. 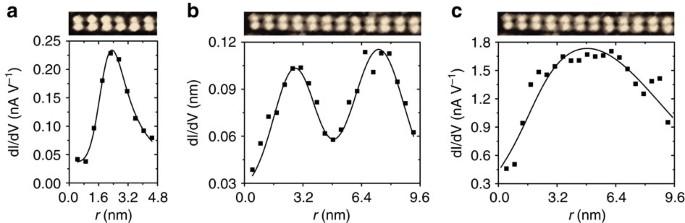Figure 4: Spatial variation of the differential conductivity of the Ir nanowires. Spatial variation of the differential conductivity at the Fermi level for an Ir nanowire with a length of 4.8 nm (a) and 9.6 nm (b). (c) Spatial variation of the differential conductivity atV=−0.275 V for the Ir nanowire from graphb.r=0 refers to one of the ends of the nanowire. The solid lines serve as a guide to the eye. STM images of the Ir nanowires are shown at the top of the graphs. The sample bias is −1 V and the tunnel current is 0.5 nA. These values were also used as set points for the I–V curves. Figure 4: Spatial variation of the differential conductivity of the Ir nanowires. Spatial variation of the differential conductivity at the Fermi level for an Ir nanowire with a length of 4.8 nm ( a ) and 9.6 nm ( b ). ( c ) Spatial variation of the differential conductivity at V =−0.275 V for the Ir nanowire from graph b . r =0 refers to one of the ends of the nanowire. The solid lines serve as a guide to the eye. STM images of the Ir nanowires are shown at the top of the graphs. The sample bias is −1 V and the tunnel current is 0.5 nA. These values were also used as set points for the I–V curves. Full size image In addition, we want to emphasize that were unable to measure any variation in the separation of nearest neighbour Ir atoms and, therefore we have to rule out the possibility that the length of the chains is stabilized by a strain effect arising from a lattice mismatch with the underlying substrate. Further, we note that the density of states oscillates very strongly. This is attributed to the slow decay of Friedel oscillations in 1D systems resulting in pronounced standing wave patterns. The low density of states near the ends of the wires suggests that the charge spill over is quite low, although we cannot exclude some contribution. Most importantly, however, is the wavelength of the oscillations of about 4.8–5 nm, which corresponds exactly with the measured preferences for certain lengths in the histogram displayed in Fig. 2 . From the observed direct match between the measured oscillations in the density of states and the preferred size of the wires, we can safely conclude that QSE are responsible for the obtained size distribution of the Ir wires on Ge(001). We note that for a 1D system, the Fermi wavelength, λ F , is directly coupled to the number density of free electrons, n 1 , at the Fermi level, irrespective of the effective mass of the electrons: λ F =4 /n 1 . With λ F =9.6 nm one arrives at n 1 =0.42 nm −1 , or the Ir atoms contribute ~1/3 electrons per wire-period to the density of states in the wires at the Fermi level. We emphasize that the Fermi wavelength is independent of the length of the Ir nanowire ( cf . equation (1)). Two last remarks are made about the histogram of the lengths of the Ir nanowires. These lengths are certainly subject to a length limitation imposed by the local width of the terraces. More important, however, is the lack of mobility of Ir atoms across the wires and their very restricted mobility along the wires because of the underlying dimer rows. This implies that it will take ‘forever’ to obtain an equilibrium distribution of Ir wire lengths. This holds both for deposition at low temperature and subsequent annealing as well as for direct deposition at high temperature. This effect is responsible for the sharp decay of the envelope at large lengths ( Fig. 2 ). We stress that strain is not responsible for this decay as it is well possible to grow much longer wires with still quantum size stabilization at low Ir coverage (see Fig. 1b ). Therefore and unfortunately, the exact size of the histogram does not provide insight in the relative energies of the various sizes. However, it is noted that a preference for smaller lengths is inhibitive for the outgrowth to micrometre lengths. We believe that this is the reason for the lack of success of our attempts to grow well-defined, almost macroscopic domains of Ir wires in contrast to the Pt- and the Au-induced wires on Ge(001). Most important in the present context is, however, a preference for lengths with multiples of ~4.8 nm, that is, six periods of 0.8 nm within the nanowire. This would indicate that the 1D analogue of equation (1) is well-satisfied and one is dealing with a combined electronic effect: QSE and constructive interference of the Friedel oscillations, which hardly decay along the short wire. The deposition and subsequent annealing of submonolayer amounts of Ir on Ge(001) result into the formation of Ir nanowires. The nanowires are defect free and have a constant width of 0.57 nm. Their periodicity along the wire corresponds to 0.8 nm. The length histogram reveals strong preferences for lengths with multiples of about 4.8 nm, that is, six elementary units of the nanowire. These nanowires are metallic and the density of states shows well-defined oscillations along the wires with a period that corresponds to the size distribution. We ascribe these findings to quantum size stabilization of selected wire lengths, very similar to well-known thickness preference in thin films. For the abundant case of nanowires with twice the elementary length, we were able to demonstrate quantum confinement of electrons: an n =2 state right at the Fermi level and an n =1 state at −275 meV from the Fermi level. Unlike the thin film case, we are able to directly probe the relevant spatial variation of the spectroscopic density of states, which allows us to pin down the electronic nature of the length preference. The nanowires have a preference for magic lengths that are integer multiples of half of the Fermi wavelength. STM and spectroscopic measurements Experiments were performed using an Omicron room temperature ultra-high vacuum STM operating at a base pressure of 5 × 10 −11 mbar. All STM and spectroscopic measurements were performed at room temperature. The current–voltage (I–V) curves are recorded with the feedback loop disabled at a set point of 0.5 nA and −1 V. Sample preparation Ge(001) samples were cut from nominally flat 3-inch single-side-polished and nearly intrinsic n -type wafers. The samples were mounted on Mo holders and contact of the samples with any other metal has been carefully avoided during the preparation. An atomically clean Ge(001) substrate was obtained by several cycles of prolonged 800 eV Ar + ion sputtering, followed by annealing the sample through resistive heating at 1,100 (±25) K [42] . The clean samples exhibited a well-ordered (2 × 1)/c(4 × 2) domain pattern (see Fig. 1a ). Subsequently, a fraction of a monolayer (0.01–0.3) of Ir was deposited on the surface by resistively heating a 99.9% pure Ir wire [23] . During evaporation the sample was kept at room temperature. After evaporation the sample was annealed at temperatures ranging from 450 to 650 K. Before placing it into the STM, the sample was cooled down to room temperature. How to cite this article: Mocking, T.F. et al . Electronically stabilized nanowire growth. Nat. Commun. 4:2387 doi: 10.1038/ncomms3387 (2013).